Kinetics of lithium peroxide oxidation by redox mediators and consequences for the lithium–oxygen cell Lithium–oxygen cells, in which lithium peroxide forms in solution rather than on the electrode surface, can sustain relatively high cycling rates but require redox mediators to charge. The mediators are oxidised at the electrode surface and then oxidise lithium peroxide stored in the cathode. The kinetics of lithium peroxide oxidation has received almost no attention and yet is crucial for the operation of the lithium–oxygen cell. It is essential that the molecules oxidise lithium peroxide sufficiently rapidly to sustain fast charging. Here, we investigate the kinetics of lithium peroxide oxidation by several different classes of redox mediators. We show that the reaction is not a simple outer-sphere electron transfer and that the steric structure of the mediator molecule plays an important role. The fastest mediator studied could sustain a charging current of up to 1.9 A cm –2 , based on a model for a porous electrode described here. The rechargeable aprotic lithium–O 2 (air) battery operates by the reduction of O 2 at the positive electrode forming Li 2 O 2 on discharge, with oxidation of Li 2 O 2 taking place on charge [1] , [2] , [3] , [4] , [5] , [6] , [7] , [8] , [9] , [10] . Li 2 O 2 is an insulating and insoluble solid [11] , [12] , [13] , [14] , [15] , [16] . Ether-based electrolytes, such as dimethoxyethane (DME) and tetra ethylene glycol dimethyl ether (tetraglyme), have been used as the basis of electrolyte solutions in most Li–O 2 cells, because of their relative stability towards reduced oxygen species. However, they cannot dissolve LiO 2 , the intermediate in the reduction of O 2 to Li 2 O 2 , 
    O_2 +  L i^ + +  e^- → LiO_2
 (1) 
    2 LiO_2 → Li_2 O_2 +  O_2
 (2) 
    LiO_2 +  Li^ + +  e^- → Li_2 O_2
 (3) resulting in LiO 2 being adsorbed on the electrode surface, and resulting in the growth of Li 2 O 2 films on the electrode, leading to low rates, low capacities and early cell death [14] , [17] . The problem is exacerbated by the formation of Li 2 CO 3 between Li 2 O 2 and carbon, the latter is usually employed as the material for the porous positive electrode [18] . Use of redox mediators (RMs) on discharge, such as 2,5-di-tert-butyl-1,4-benzoquinone (DBBQ), which are reduced at the electrode surface on discharge and then go on to reduce O 2 to Li 2 O 2 in solution, can help to mitigate these problems, but result in the formation of Li 2 O 2 disconnected from the electrode surface and therefore electronically isolated during charging [19] . This introduces the need for a redox mediator to be employed on charging that can oxidise Li 2 O 2 [20] , [21] , [22] , [23] , [24] , [25] , [26] , [27] , [28] , [29] , [30] , [31] , [32] , [33] . Such mediators are molecules capable of oxidation at the surface of the pores in the porous positive electrode on charging and then transfer of holes to the electronically isolated Li 2 O 2 particles within the pores. As a result, Li 2 O 2 is oxidised and O 2 released, the mediator molecule being reduced in the process and returning to the electrode surface for the cycle to be repeated. Suitable oxidation mediators must have a redox potential above that for O 2 /Li 2 O 2 : 2.96 V vs. Li + /Li, a sufficiently high heterogeneous rate constant for electron transfer at the electrode surface to support the required charging rates, a highly reversible redox process such that the cycle may be carried out many times, and of course not only be capable of oxidising Li 2 O 2 , but with a sufficiently high rate to sustain the required charging current [34] . Stability of the mediators, especially on long-term cycling, is also an important challenge and recent work has considered the design of more stable redox mediators for cycling [22] ; however, very little is known about the factors affecting the reaction between oxidation mediators and Li 2 O 2 . It is often assumed that a mediator with a high redox potential has fast kinetics for the oxidation of Li 2 O 2 , but this is not necessarily so [33] . Alternatively, the kinetics of Li 2 O 2 oxidation by a mediator could be linked to the kinetics of its own redox process, but this would only be the case if both were outer-sphere electron transfer processes. Importantly, little experimental evidence exists about the kinetics of Li 2 O 2 oxidation by redox mediators, yet their use and such kinetics are crucial to the operation of the Li–O 2 cell. Here, we investigate the kinetics of Li 2 O 2 oxidation by several classes of redox mediators, which differs in the E o (standard redox potential) and k o (standard heterogeneous electron transfer rate constant) values, to ascertain the factors that control the rate of Li 2 O 2 oxidation by the mediators. Apparent rate constants ( k app ) of mediators Apparent rate constants ( k app ) for Li 2 O 2 oxidation by the redox mediators were determined using scanning electrochemical microscopy (SECM). Details of the cell and procedures used are given in the Methods section. In brief, SECM feedback approach curves at a Li 2 O 2 disk, composed of a pressed pellet of commercial Li 2 O 2 with a diameter of 12 mm, were recorded and apparent rate constants, k app , for Li 2 O 2 oxidation were obtained by fitting to the theoretical feedback approach curves developed by Cornut et al. [35] , [36] , [37] . When recording an approach curve, the SECM tip was held at a sufficiently positive potential such that a steady-state current was obtained for the oxidation of the redox mediator. The tip approaches the Li 2 O 2 disk and at small separation distances, the mediator oxidised at the tip diffuses to the Li 2 O 2 disk where it oxidises Li 2 O 2 , regenerating itself and contributing to a feedback loop, while concurrently, diffusion of the mediator to the tip is blocked by the surface. 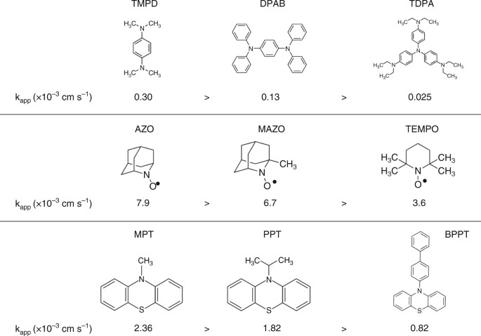Fig. 1 Structures of the oxidation mediators and their kinetics of Li2O2oxidation. Comparison of the apparent rate constants (kapp) for the reaction between the redox mediators and Li2O2grouped by structure The balance of the two alter the current at the SECM tip, i T , and the faster the kinetics of Li 2 O 2 oxidation by the mediator the greater the current, see Supplementary Figure 1 . As we do not know the mechanism by which the mediators oxidise the lithium peroxides surface, we can only obtain an apparent rate constant ( k app ) based on the feedback response; however, this provides a comparison between the different mediators and indicates the overall rate capability. Fig. 1 shows the oxidation mediators studied. They are in three classes, amines, nitroxy and thiol compounds, chosen because they are classes of compounds known to exhibit reversible redox processes and include several of the compounds that have been used as oxidation mediators in Li–O 2 cells, such as tris[4-(diethylamino)phenyl]amine (TDPA), 2,2,6,6-tetramethyl-1-piperidinyloxy (TEMPO) and 10-methylphenothiazine (MPT) [20] , [21] , [22] . k app for Li 2 O 2 oxidation by the mediators are presented in Supplementary Table 1 . The standard redox potential, E o , and standard heterogeneous electron transfer rate constant, k o , were measured for each mediator using cyclic voltammetry, as described in the Methods section. The diffusion coefficients, D , were obtained from the steady-state current at an ultramicroelectrode (UME), also as described in the Methods section. The values for each of the three parameters are also given in Supplementary Table 1 . Three additional mediators, tetrathiafulvalene (TTF), ferrocene (FC) and 5,10-dimethylphenazine (DMPZ), which do not belong to the above three classed, but have been commonly used as oxidation mediators, were also studied and are listed in Supplementary Table 1 [23] , [24] , [38] . The standard redox potentials are all positive for the O 2 /Li 2 O 2 reaction. The diffusion coefficients vary by no more than a factor of 3. The k o for the mediators themselves are all relatively high, ranging from 0.007 to 0.078 cm s –1 , sufficiently so to support an areal current density over 200 mA cm −2 at an overpotential of 60 mV, based on the true surface area of the pores and therefore more than sufficient to sustain an areal current density suitable for a Li–O 2 cell. Of course, this does not take into account the kinetics of Li 2 O 2 oxidation required to sustain the current, which will be discussed below after the presentation of the rates of Li 2 O 2 oxidation. The assumptions regarding the porous cathode structure and the approach used to make this estimate are described in the Supplementary Note. Fig. 1 Structures of the oxidation mediators and their kinetics of Li 2 O 2 oxidation. Comparison of the apparent rate constants ( k app ) for the reaction between the redox mediators and Li 2 O 2 grouped by structure Full size image Before considering the kinetics of the mediator oxidation in more detail, we first determine the surface composition of the disk and the possibility of passivation with, for example, Li 2 CO 3 . A disk of Li 2 O 2 was immersed in 1 M LiTFSI in tetraglyme for 3 h and then examined by time of flight secondary ion mass spectrometry (TOF-SIMS), alongside a disk that was not exposed to the electrolyte solution. As shown in Fig. 2 , for both disks, the major peaks are from Li 2 O 2 + , with the secondary peaks being ascribed to Li 2 CO 3 . These results show that although there is some Li 2 CO 3 , even on the surface of the pristine disk, a significant proportion of the surface remains as Li 2 O 2 even after 3 h of exposure to the electrolyte, confirming that the disk is suitable for the SECM measurements. Note that the sensitivity of TOF-SIMS to different species varies, consequently it is not possible to quantify the relative amounts of Li 2 O 2 and Li 2 CO 3 by simply comparing the areas under the peaks. Instead, the disk was etched until the signal from Li 2 O 2 was constant, therefore corresponding to the bulk peroxide, i.e., 100% Li 2 O 2 . Comparing this signal with that for Li 2 O 2 at the surface indicated that approximately 35% of the disk surface was Li 2 O 2 . Fig. 2 TOF-SIMS of Li 2 O 2 disks before and after treating with electrolyte of 1 M LiTFSI in tetraglyme. Both Li 2 O 2 disks show signal of Li 2 O 2 + and Li 2 CO 3 + whereas the Li 2 CO 3 disk shows little signal of Li 2 O 2 + , confirming the presence of Li 2 O 2 on the surface of disk after treating with the electrolyte Full size image A disk of Li 2 CO 3 was investigated with SECM using TEMPO as the oxidation mediator, as it has a sufficiently high potential to oxidise Li 2 CO 3 and shows fast kinetics with the Li 2 O 2 disk. 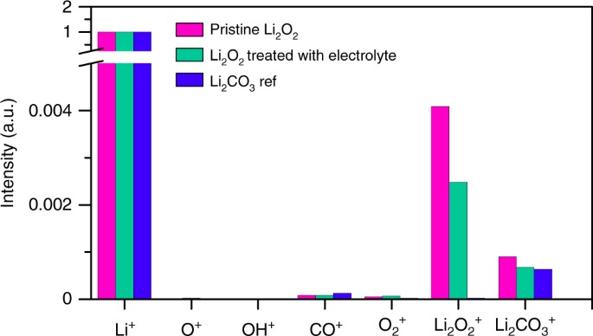Fig. 2 TOF-SIMS of Li2O2disks before and after treating with electrolyte of 1 M LiTFSI in tetraglyme. Both Li2O2disks show signal of Li2O2+and Li2CO3+whereas the Li2CO3disk shows little signal of Li2O2+, confirming the presence of Li2O2on the surface of disk after treating with the electrolyte The results are shown in Supplementary Figure 2 . The k app for oxidation of Li 2 CO 3 by TEMPO is four orders of magnitude lower than the data collected on the Li 2 O 2 disk, indicating that even for mediators with sufficiently high potentials the contribution of Li 2 CO 3 oxidation to the k app is very small. The dominant reaction for the range of mediators studied here, even taking account of partial coverage by Li 2 CO 3 , is oxidation of Li 2 O 2 . It has been reported previously by us and by others that several of the redox mediators used in Li–O 2 cells to date exhibit some degree of decomposition [24] , [39] , [40] , [41] . 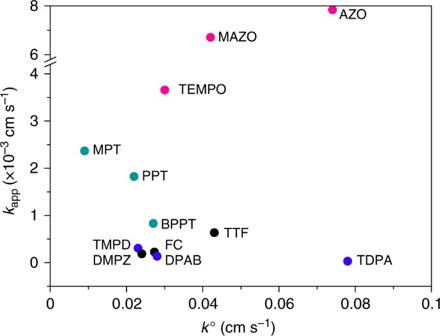Fig. 3 Dependence of the apparent rate constant,kapp, on the heterogeneous electron transfer rate constant,ko, of the mediators. Amines, nitroxy and thiol compounds are marked in blue, red and green Assembling a cell with commercial Li 2 O 2 and the oxidation mediators TTF and AZO, and then charging to a capacity of ∼ 1 mAh results in notable decomposition of TTF and AZO as seen by 1 HNMR of the electrolyte, see Supplementary Figure 3 . In the SECM experiments, only a small amount of charge, ∼ 1 nAh, is passed, therefore the fraction of mediator that is decomposed is negligible. Inner-sphere process for mediator oxidising Li 2 O 2 To explore the possible correlations between k app and the electrochemical parameters of the redox mediators, E o and k o , plots of k app vs. k o and E o and are presented in Figs. 3 and 4 , respectively. There is no apparent dependence of k app on k o , Fig. 3 . 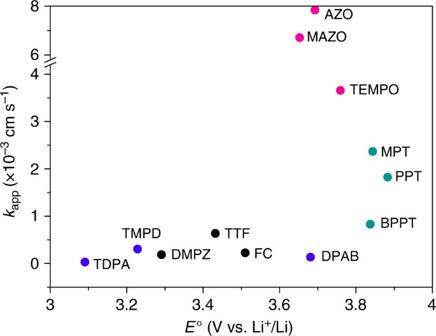Fig. 4 Dependence of the apparent rate constant,kapp, on the redox potential,Eo, of the mediators. Amines, nitroxy and thiol compounds are marked in blue, red and green The values of k o for the different redox mediators appear independent of the nature of the electrode used to measure them, as demonstrated by measuring these values at Au and glassy carbon electrodes, see Supplementary Figure 4 and Methods section, consistent with the RM + /RM reactions occurring by outer-sphere electron transfer. If the oxidation of Li 2 O 2 was also an outer-sphere electron transfer reaction, then k app would be proportional to k o of the redox mediator (and hence the reorganisation energy of the RM and surrounding solution), or the rate of the reaction Li 2 O 2 → Li 2 O 2 + + e − . Since there is no dependence of k app on k o , the former cannot be true. If the rate was limited by the electron transfer kinetics associated with the Li 2 O 2 , then k app would be invariant, which again is not the case. We conclude that oxidation of Li 2 O 2 by the redox mediators is mainly an inner-sphere process, i.e., involves adsorption of the mediator on the peroxide surface. The values for k app are one order of magnitude smaller than the corresponding k o values, indicating that the reaction of mediators oxidising Li 2 O 2 is most likely to be the rate determining step of the entire charge process. This will particularly be true towards the end of charge when the surface area of the remaining Li 2 O 2 is low. We estimate that a k app from 2.5 × 10 –5 to 7.9 × 10 –3 cm s –1 in a Li–O 2 cell with a porous cathode filled with Li 2 O 2 would provide an areal current density of 108 mA cm –2 to 1.9 A cm –2 using the same model for the porous cathode as above. The details are described in the Supplementary Note and Supplementary Figure 5 . Although we note that this equivalent charging current varies with consumption of Li 2 O 2 , it is sufficient to sustain the charging process, even for some of the slowest oxidation mediators investigated here. Fig. 3 Dependence of the apparent rate constant, k app , on the heterogeneous electron transfer rate constant, k o , of the mediators. Amines, nitroxy and thiol compounds are marked in blue, red and green Full size image Fig. 4 Dependence of the apparent rate constant, k app , on the redox potential, E o , of the mediators. Amines, nitroxy and thiol compounds are marked in blue, red and green Full size image Turning to the plot of k app vs. E o , Fig. 4 , it appears that the highest rates are observed for mediators with potentials above ∼ 3.6 V. However, potential per se is not the explanation for the high rate, as there are examples of mediators with a high potential but low rate, e.g., BPPT. From the experiment on the Li 2 CO 3 disk using TEMPO, we know higher rates at high potentials are not due to the onset of Li 2 CO 3 oxidation contributing to the overall surface oxidation kinetics. Different crystal facets of Li 2 O 2 will have different oxidation potentials [42] . Mediators operating at higher potentials could oxidise these higher potential facets and hence access a greater Li 2 O 2 surface area. However, the fact that the rates vary for different mediators above 3.6 V and several high potential mediators have relatively low k app suggests that this alone cannot be the reason for high rate mediators having a relatively high potential. As discussed below, we believe an important factor controlling the rate of the mediators is the nature of the oxidising centre and the degree of its steric hindrance. Considering the molecules presented in Fig. 1 and the k app values shown in the figure, it is evident that the nitroxy radicals exhibit the fastest rates of Li 2 O 2 oxidation. The thiol group also provides a high rate, in contrast to the amines that are all low rate. The chemistry of the redox centre appears to be an important factor for controlling the rate of oxidation, probably due to the interaction with Li 2 O 2 surface. The oxidation rates decrease when the redox centre of the molecule is surrounded by bulky groups, Fig. 1 . This suggests that a key factor influencing the kinetics of Li 2 O 2 oxidation is the steric hindrance as the molecule approaches the surface of Li 2 O 2 . The fastest kinetics is exhibited by 2-azaadamantane- N -oxyl (AZO), 7.9 × 10 –3 cm s –1 , which has the most exposed redox centre of all the redox mediators studied here. This observation is in accord with the lack of evidence for an outer-sphere reaction and provides direct evidence for Li 2 O 2 oxidation proceeding by an inner-sphere mechanism. In conclusion, we have measured the rate constants for the oxidation of Li 2 O 2 particles by a series of molecular mediators spanning standard redox potentials, E o from 3.1 to 3.9 V and standard heterogeneous rate constants for electron transfer, k o from 0.007 to 0.078 × 10 –3 cm s –1 . The surface of Li 2 O 2 particles in a typical electrolyte solution, LiTFSI in tetraglyme, is partially covered by Li 2 CO 3 , but the rate of Li 2 CO 3 oxidation, a mediator that operates at 3.8 V, TEMPO, is four orders of magnitude lower than for Li 2 O 2 , therefore Li 2 O 2 oxidation dominates. There is no correlation between the variation of k o , the standard heterogeneous rate constant at the electrode surface for the mediators, and the rate of Li 2 O 2 oxidation by the mediators, indicative of this not being an outer-sphere electron transfer process at the Li 2 O 2 surface. There is evidence of Li 2 O 2 oxidation rates depending on the nature of the oxidising molecule. Nitroxy radicals, especially those with low steric hindrances of access to the Li 2 O 2 surface, exhibit the highest rates. Nevertheless, the mechanism of Li 2 O 2 oxidation by molecular oxidants is still not well understood, and such understanding will be important in order to inform the design of optimised oxidation mediators. All mediators studied display kinetics sufficient to enable relatively high rates within a battery, charging current density exceeding 100 mA cm –2 . A mediator with a k app of 7.9 × 10 –3 cm s –1 can sustain an areal current density of up to 1.9 A cm –2 , based on the same model. It is important to note that stability is still a challenge for the Li–O 2 battery and here we observe significant mediator decomposition when passing large amounts of charge. More stable electrolytes and mediators are required to minimise side reactions and hence improve cycleability. Materials preparation Li 2 O 2 and Li 2 CO 3 disks were obtained by pressing Li 2 O 2 powder (Aldrich) and Li 2 CO 3 powder (Aldrich) with a die set in an Ar-filled glove box. Disks of 13 mm diameter and ∼ 1 mm of thickness were prepared and served as substrate. A Au microelectrode (diam. 25 μm, CHI) served as an SECM probe tip. Prior to measurement, the Au tip was polished with a microelectrode beveller (Sutter) and checked with a microscope. A silver wire reference electrode (RE) and a platinum counter electrode (CE) were used. 2,2,6,6-tetramethyl-1-piperidinyloxy (TEMPO), 2-azaadamantane- N -oxyl (AZO), 1-methyl-2-azaadamantane- N -oxyl (MAZO), tris[4-(diethylamino)phenyl]amine (TDPA), 1,4-bis(diphenylamino)benzene (DPAB), N , N , N ′, N ′-tetramethyl-p-phenylenediamine (TMPD), 10-methylphenothiazine (MPT), 10-isopropylphenothiazine (PPT), 10-(4-biphenylyl)phenothiazine (BPPT), tetrathiafulvalene (TTF), ferrocene (FC) and 5,10-dimethylphenazine (DMPZ) are from Aldrich. 10 mM redox mediators are dissolved in 100 mM LiTFSI–tetraglyme electrolyte for electrolyte solution. A Swagelok cell was assembled as reported previously [40] , using a piece of gas diffusion layer electrode (GDL) as the positive electrode. A lithium super ionic conductor disc (LiSICON, Ohara) was used to protect Li metal as the negative electrode. A Li 2 O 2 disk was placed between the GDL and the LiSICON essentially placing the cell in a discharged state. TTF and AZO were chosen as the oxidation mediators. The cell was charged by holding at 3.4 V for TTF and 3.7 V for AZO until 1 mAh charge passed prior to further chemical characterisations. For NMR analysis, the electrodes and separators were rinsed with 0.7 ml of CDCl 3 , and measurements were recorded on a Bruker spectrometer (400 MHz). Electrochemical measurements SECM experiments were performed with SECM bipotentiostat (CHI 920) in an Ar-filled glovebox. Prior to kinetics measurement, the NG factor of Au tip was determined by approaching a completely insulating surface and fitting the negative approach curve. The data processing and fitting process were described elsewhere [35] , [36] , [37] . A dimensionless rate constant, κ , was obtained by data fit, which equals to k app r o / D , where r 0 is the radius of tip and D is the diffusion coefficient of redox mediators. D of various mediators were determined by measure steady-state current of a Au microelectrode with known radius r 0 , according to i ss =4 nFDr o C . The redox potential and heterogeneous electron transfer rate constants k o of redox mediators itself were determined using cyclic voltammetry(CV) measurements. The redox potential is determined by the centre of two redox peaks, which is measured in a 100-mM LiTFSI–tetraglyme solution with 10 mM of various mediators at a Au electrode. Partially charged LiFeO 4 (LFP) protected by a glass frit served as an RE and it gave a potential of 3.45 V vs. Li + /Li as reported previously. A platinum wire served as a CE. The details of k o measurement are described elsewhere [43] . Briefly, CVs were recorded at various scan rates, ranging from 0.05 to 10 V s –1 . Ψ , a function of CV peaks separation, was plotted vs. root of scan rate and a linear fit was applied. k o was obtained from the slope of linear fit. The k o measurement was carried out at both Au and glassy carbon (GC) WEs. Due to the non-negligible resistance of ether-based electrolytes, an Ohmic overpotential correction was applied to account for the uncompensated resistence during  CV measurements and a silver wire RE was used. Characterisations For the surface characterisations, the Li 2 O 2 disk was immersed in 1 M LiTFSI–tetraglyme solution for 3 h prior to XPS and TOF-SIMS experiments. Both pristine disk and treated disk were characterised in an air-sensitive holder. To measure the TOF-SIMS of bulk Li 2 O 2 , the data were recorded after 2 min etching. Data availability The data that support the findings of this study are available from the corresponding author upon reasonable request. Background data has been deposited in the Oxford Research Archive (ORA) at: https://ora.ox.ac.uk/objects/uuid:c23a0cc0-55b5-455f-bb68-a14d8ea2e3bc .